Nanoantenna-enhanced ultrafast nonlinear spectroscopy of a single gold nanoparticle Optical nanoantennas, just like their radio-frequency equivalents, enhance the light-matter interaction in their feed gap. Antenna enhancement of small signals promises to open a new regime in linear and nonlinear spectroscopy on the nanoscale. Without antennas especially the nonlinear spectroscopy of single nanoobjects is very demanding. Here we present the first antenna-enhanced ultrafast nonlinear optical spectroscopy. In particular, we use the antenna to determine the nonlinear transient absorption signal of a single gold nanoparticle caused by mechanical breathing oscillations. We increase the signal amplitu-de by an order of magnitude, which is in good agreement with our analytical and numerical models. Our method will find applications in linear and nonlinear spectroscopy of single nanoobjects, especially in simplifying such challenging experiments as transient absorption or multiphoton excitation. Nanoobjects with a size between 1 and 100 nm show fascinating properties which deviate strongly from bulk behaviour. The plasmon resonance of metal nanoparticles and the electron confinement in quantum dots are prominent examples. However, even with the best preparation methods, the individual objects differ from each other in size, shape or local environment, rendering necessary single-object experiments [1] . As the light-matter interaction strength scales with the number of electrons involved, the signals of an individual nanoobject become very weak. Especially, the nonlinear signals, which are already weak for bulk material, become difficult if not impossible to detect [2] , [3] , [4] , [5] , [6] , [7] , [8] , [9] . A resonant optical nanoantenna [10] , [11] that concentrates the optical field on the individual nanoobject promises enhancement of such weak nonlinear signals ( Fig. 1 ). In previous work, nonlinear effects were used to characterize the antenna itself [12] , [13] . Here we use the resonant antenna for spectroscopy and demonstrate nanoantenna enhancement of the ultrafast transient transmission of a single metal nanodisc [6] . This transient transmission spectroscopy is a nonperturbative optical method to investigate mechanical properties at the nanoscale. It is particularly suited to test our concept. A pump-pulse triggers acoustical vibrations. The oscillations lead to a periodic variation of the particle size and of the plasma frequency by the electron density. This modifies in turn the dielectric function [14] , [15] . In this way, we determine the oscillation eigenfrequency of a tiny nanodisc and Young's modulus at the nanoscale [16] . 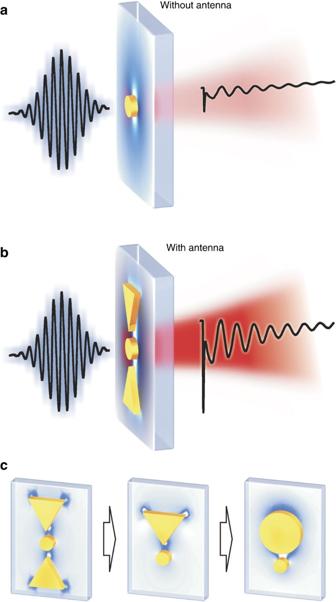Figure 1: Illustration of signal enhancement using a resonant optical nanoantenna. (a) A single nanoobject of few nanometres in size is probed by an ultrashort laser pulse. The resulting nonlinear response is extremely weak, but carries information about the physical processes. (b) An optical nanoantenna (represented by the bowtie structure) enhances the nonlinear response of the nanoparticle by increasing the light-matter interaction at the nanofocus. (c) For the demonstration of this effect, we chose a structure for which we can model reliably both the electromagnetic as well as the mechanic properties. More evolved antennas promise an even larger enhancement and offer degrees of freedom to adjust the antenna to special needs. Figure 1: Illustration of signal enhancement using a resonant optical nanoantenna. ( a ) A single nanoobject of few nanometres in size is probed by an ultrashort laser pulse. The resulting nonlinear response is extremely weak, but carries information about the physical processes. ( b ) An optical nanoantenna (represented by the bowtie structure) enhances the nonlinear response of the nanoparticle by increasing the light-matter interaction at the nanofocus. ( c ) For the demonstration of this effect, we chose a structure for which we can model reliably both the electromagnetic as well as the mechanic properties. More evolved antennas promise an even larger enhancement and offer degrees of freedom to adjust the antenna to special needs. Full size image Currently, different kinds of antenna structures are under development in the optical regime, ranging from simple dipoles to complex Yagi-Uda antennas [12] , [17] , [18] , [19] , [20] . In our experiment, we use a polarization-insensitive dipole antenna, that is, a plasmonic nanodisc of 70 nm diameter ( Fig. 2a ). As the nanoobject under investigation we pick a nanodisc of smaller diameter (40 nm) whose linear optical scattering signals are already very weak and transient absorption is nearly impossible to detect. We find a transient signal that arises from the coupled antenna-nanoparticle structure. Compared with the nanoparticle alone, the signal is increased by an order of magnitude, in good agreement with our simulations. By changing the polarization direction of the probe beam, we can selectively switch on and off the antenna enhancement. We expect our method to find applications in linear and nonlinear spectroscopy of nanoobjects, ranging from single-protein binding events [21] via nonlinear tensor elements [22] to the limits of continuum mechanics [23] . 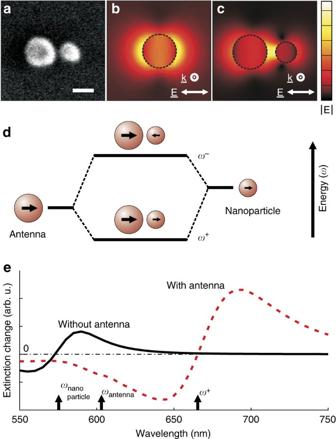Figure 2: Basic concept of an antenna for a plasmonic particle. (a) Scanning electron microscopy picture of the structure: nanoantenna (disc diameter 70 nm) separated from the nanoparticle under investigation (disc diameter 40 nm) by a gap of 15 nm. Both elements are made by electron beam lithography out of gold (height 30 nm) on a glass substrate (scale bar, 50 nm). (b,c) Absolute value of the electric field in the top plane of the structure. The wavelength is in each case adjusted to the resonance. (d) A coupled antenna-nanoobject system has new eigenmodes, determined by plasmon hybridization. (e) The change in extinction of a coupled system (dashed line) by varying the nanoparticle's plasma frequency is enhanced and red shifted, compared with the case of an uncoupled nanoparticle (solid line). Figure 2: Basic concept of an antenna for a plasmonic particle. ( a ) Scanning electron microscopy picture of the structure: nanoantenna (disc diameter 70 nm) separated from the nanoparticle under investigation (disc diameter 40 nm) by a gap of 15 nm. Both elements are made by electron beam lithography out of gold (height 30 nm) on a glass substrate (scale bar, 50 nm). ( b , c ) Absolute value of the electric field in the top plane of the structure. The wavelength is in each case adjusted to the resonance. ( d ) A coupled antenna-nanoobject system has new eigenmodes, determined by plasmon hybridization. ( e ) The change in extinction of a coupled system (dashed line) by varying the nanoparticle's plasma frequency is enhanced and red shifted, compared with the case of an uncoupled nanoparticle (solid line). Full size image Modelling of the antenna effect The optical properties of a gold nanodisc are dominated by a dipolar plasmon resonance. Close to the resonance, the optical near-field around the disc shows a dipolar pattern with two regions of high field intensity ( Fig. 2b ). These hot spots function similar to a nanolens by concentrating the field in a small volume [24] . A variation of the dielectric function in this volume will have a large influence on the transmitted field. This is the antenna effect we exploit for signal enhancement. In our case, the perturbation of the antenna by the nanoobject is not negligible. Both antenna and nanoobject together form a coupled system with common eigenmodes and an altered field distribution ( Fig. 2c ). The common eigenmodes of the coupled system can be described in the plasmon hybridization picture [25] , [26] by dipole–dipole interactions. These coupled modes are the symmetric ( ω + ) and antisymmetric ( ω − ) combination of the original modes ( Fig. 2d ). If antenna and nanoobject were equal in size, the symmetric mode ω + would carry all the oscillator strength. In our case, both modes are optically active. However, the high-energy antisymmetric mode ω − is shifted into the d-band absorption of gold and thus damped out. For a polarization direction perpendicular to the symmetry axis, the dipole coupling and thus the mode splitting is reduced. The strong, symmetric mode becomes the blue-shifted mode and is damped because of absorption. In the uncoupled case, a pump-induced variation of the plasma frequency of the nanoparticle shifts the extinction spectrum of the nanoparticle only, resulting in a dispersive feature in the differential spectrum at the plasmon resonance frequency ω nanoparticle of the nanoparticle (solid line in Fig. 2e ). When antenna and nanoparticle form a coupled system, the influence of the dielectric function of the particle is amplified by the larger oscillator strength of the coupled system. This results in a larger variation of the extinction (dashed line in Fig. 2e ) now located at the coupled antenna mode ω + . Thus, a successful operation of the antenna is characterized by a red shift and an amplification of the nonlinear signal of the particle. Ultrafast spectroscopy of a single antenna In the following, we verify these theoretical predictions by ultrafast pump-probe spectroscopy (Methods) [6] , [16] . A laser pulse is focused onto a single antenna-nanoobject pair. The pulse heats up the electron gas and subsequently the lattice. On a picosecond timescale this launches mechanical breathing oscillations of the particles. The periodic variation of the particle volume causes a transient time-dependent extinction. After a variable time delay, a probe pulse measures the pump-induced relative transmission variation Δ T / T in the 10 −6 range. By varying the time delay between pump- and probe-pulse we acquire mechanical oscillation traces. In the simulations, we are able to vary the optical properties of the nanoparticle only. However, in the experiment, the pump-pulse excites the nanoparticle and the antenna. Consequently, both start to oscillate. 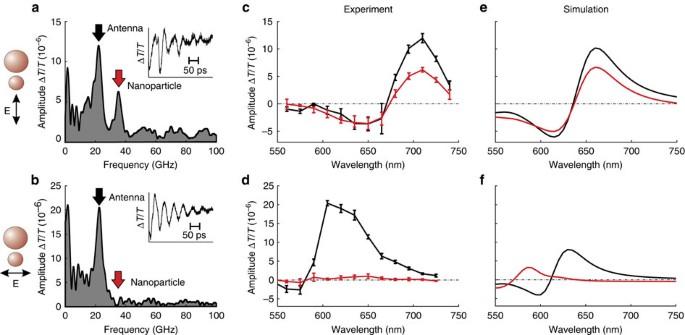Figure 3: Experimental results compared with simulations. The polarization of the probe light determines the coupling strength between antenna and nanoparticle. The upper row of plots (a,c,e) shows the strong coupling case, lower row (b,d,f) the weak coupling control experiment. The response of the nanoparticle and the antenna are drawn in red and black, respectively. The insets inaandbgive an example for transient transmission traces, monitoring the mechanical oscillation of the nanoparticles at their maximum signals. The corresponding mechanical spectra (a,b) show always the antenna mode (22 GHz), but only in the strong coupling case (a) also the nanoparticle mode at 36 GHz. (c,d) Oscillation amplitude of both modes as function of probe wavelength as mean of six consecutive measurements. The error bars give the standard deviation. The line is a guide to the eye. (e,f) Numerical simulations of the oscillation amplitude spectrum. The inset of Figure 3a shows an example for the measured oscillation trace at 710 nm probe wavelength. Its Fourier transform ( Fig. 3a ) shows two distinct peaks at 22 and 36 GHz. We assign the lower frequency mode to the antenna and the higher mode to the nanoparticle based on measurements of individual single discs of different size. The Fourier decomposition thus allows us to distinguish between the mechanical signals from antenna and nanoparticle. In the following, we plot the amplitudes of these two Fourier components as a function of probe wavelength. Figure 3: Experimental results compared with simulations. The polarization of the probe light determines the coupling strength between antenna and nanoparticle. The upper row of plots ( a , c , e ) shows the strong coupling case, lower row ( b , d , f ) the weak coupling control experiment. The response of the nanoparticle and the antenna are drawn in red and black, respectively. The insets in a and b give an example for transient transmission traces, monitoring the mechanical oscillation of the nanoparticles at their maximum signals. The corresponding mechanical spectra ( a , b ) show always the antenna mode (22 GHz), but only in the strong coupling case ( a ) also the nanoparticle mode at 36 GHz. ( c , d ) Oscillation amplitude of both modes as function of probe wavelength as mean of six consecutive measurements. The error bars give the standard deviation. The line is a guide to the eye. ( e , f ) Numerical simulations of the oscillation amplitude spectrum. Full size image In the upper row of Figure 3 , the probe pulse is polarized along the symmetry axis of the structure (strong antenna-nanoparticle coupling), and in the lower row perpendicular to it (weak coupling). In the first case ( Fig. 3c ), the oscillation amplitude spectra of antenna and nanoparticle are similar in spectral shape and position. Both follow the coupled antenna-nanodisc mode. These findings agree well with a dipole–dipole coupling picture ( Fig. 2d,e ), in which the mechanical oscillation of the smaller nanodisc causes a high-frequency modulation of the coupled mode extinction signal. Full numerical simulations ( Fig. 3e , calculation details in Methods) are in good agreement. All spectral features and signal amplitudes, as well as the amplitude ratio between antenna and nanoparticle signal are well reproduced. To perform a control experiment, we turn to the weak coupling case for a probe polarization perpendicular to the symmetry axis. We see a significant change of the detected mechanical oscillation signal as plotted in the inset of Figure 3b for a probe wavelength of 605 nm. The corresponding Fourier amplitudes show just one peak, located at the mechanical eigenmode frequency of the nanoantenna at 22 GHz. The 36 GHz signal of the small nanoparticle is not recognizable, although the pump excitation process is identical for both measurements. This behaviour proves the concept of our resonant antenna enhancement based on polarization-dependent plasmonic coupling. Mechanical coupling of the nanoparticle to the antenna by the substrate would be independent of the probe polarization. Plotting the mechanical oscillation signal of antenna and nanoparticle versus the probe wavelength ( Fig. 3d ), a clear change has taken place when compared with the strong coupling polarization ( Fig. 3c ). The oscillation amplitude spectrum of the antenna is still clearly observable and located around the uncoupled antenna resonance. The oscillation signal of the small nanoparticle vanishes almost completely. The numerical model ( Fig. 3f ) catches the essence: we observe a nearly undisturbed signal from a single antenna and a very weak nanoparticle signal. Figure 3c,d demonstrates clearly that we can turn the antenna enhancement on and off by switching the probe polarization appropriately. Efficiency and spectral response are two fundamental features of an antenna. To describe these features we have to compare the response of an antenna-enhanced nanoparticle with that of a single nanoparticle of the same size and shape. Because of slight variations in size, crystallinity, and damping, the oscillation amplitudes vary between nominally identical nanoparticles. Nanodiscs of 40 nm diameter, as used in combination with the antenna, are at the limit of our current detection capabilities. We increased the pump power and measured several discs of that size ( Supplementary Figs S1 and S2 ). For the comparison, we select a disc in the centre of the Gaussian amplitude distribution. 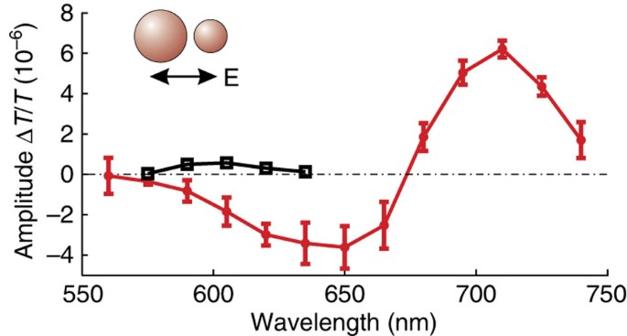Figure 4: Enhancement of the oscillation signal by the nanoantenna. The weak signal measured on a single disc with 40 nm diameter (black squares) compared with the signal amplified by the antenna structure (red dots). As predicted we find a red shift and an enhancement of the signal amplitude. The error bars give the standard deviation of six consecutive measurements. In the case of the nanoparticle without antenna, the error bars are smaller than the symbols. The lines are guides to the eye. The oscillation amplitude spectrum is plotted as squares in Figure 4 . It is obvious that the strongest signal is located around the highest gradient of the plasmon resonance where the biggest extinction change is expected. This reference signal can be compared with the antenna-enhanced signal (dots in Fig. 4 ), which was already shown in Figure 3c . The feature is red shifted and located around the plasmon resonance of the coupled antenna. The maximum amplitude is about a factor of ten larger than the signal from the nanoparticle without an antenna. This mechanical oscillation signal is the strongest oscillation that we have ever measured in such a small single nanoparticle. As the antenna concentrates also the pump field on the nanoparticle, stronger mechanical oscillations are launched when the antenna is present. By numerical simulations, we estimate an increase by a factor of about 3, so that in the present case pump and probe enhancement contribute equally to the total signal enhancement. Figure 4: Enhancement of the oscillation signal by the nanoantenna. The weak signal measured on a single disc with 40 nm diameter (black squares) compared with the signal amplified by the antenna structure (red dots). As predicted we find a red shift and an enhancement of the signal amplitude. The error bars give the standard deviation of six consecutive measurements. In the case of the nanoparticle without antenna, the error bars are smaller than the symbols. The lines are guides to the eye. Full size image We envision that our antenna-enhancement technique opens up new possibilities for linear and nonlinear spectroscopy on the nanoscale. Not only plasmonic nanoparticles, but also optically less active nanoobjects such as dielectric particles and biomolecules will detune the optical antenna [27] . Their static linear as well as their ultrafast nonlinear response becomes thus accessible in the optical far-field. We expect our method not only to simplify the research on single molecules or quantum dots, but also to open the way for modern antenna-enhanced sensing and ultrafast telecommunication applications. Experimental setup and data analysis The output of a Ti:sapphire laser was used as pump pulses (wavelength 800 nm, duration 200 fs, repetition rate 76 MHz). Probe pulses were generated by feeding part of the pump pulses into a white-light fibre and selecting a 5-nm spectral interval. This results in pulses of 2 ps duration tunable between 530 and 750 nm. After setting the polarization state, both pump and probe pulses are coupled into a home-built sample-scanning confocal microscope and focused with a numeric aperture (NA) of 0.95 objective on the sample surface. The transmitted light is collected using a NA=1.3 oil immersion objective and detected by a balanced photodiode after filtering out the pump light. More details can be found in the Supplementary Figure S3 and Supplementary Table S1 . Differential transmission traces were measured as a function of pump-probe delay. To extract the oscillatory part, an exponential decay was fitted and subtracted, removing the thermal background signal. The complex-valued Fourier transform was calculated for each trace. The mechanical mode spectra ( Fig. 3a,b ) show the absolute Fourier values. The mechanical oscillation signal of a given mode has a wavelength-independent phase relative to the pump pulse, as all probe wavelengths monitor the same mechanical oscillation [14] , [15] , causing a wavelength-independent phase of a mode's complex-valued Fourier component (for details see Supplementary Figs S4 and S5 ). This is used to check the quality of the data and to retrieve the sign in the amplitude spectrum Figures 3c,d and 4 . Numerical simulations For the numerical simulations, we used a Null-Field Method [28] and a Finite-Element Method [29] , which give nearly equal results. We approximated our structure by gold nanodiscs in an homogeneous medium. For a single disc, an effective index of refraction of n =1.42 yields a good agreement between measured and calculated dark field scattering spectra. However, the mode splitting of a coupled disc pair is underestimated in this model. The step in index of refraction at the interface seems to be more important in near-field coupling. This explains the differences in spectral position between experiment and simulation in Figure 3 . For the differential transmission data, we took the difference between an unperturbed sample and a sample in which both the nanoparticle's dielectric function and its size were changed. For the size change of the particle, we use an isotropic thermal expansion model, and a temperature variation proportional to the Joule heating of the pump pulse in the particle. The change of the dielectric properties is modelled in our wavelength range by a Drude model. The size-induced variation of the electron density results in a variation of the plasma frequency [30] . The d-band absorption is extracted from Johnson and Christy data [31] and kept constant. This renders our simulations below a probe wavelength of about 600 nm unreliable. How to cite this article: Schumacher, T. et al . Nanoantenna-enhanced ultrafast nonlinear spectroscopy of a single gold nanoparticle. Nat. Commun. 2:333 doi: 10.1038/ncomms1334 (2011).